Dynamic catch of a Thy-1–α5β1+syndecan-4 trimolecular complex Cancer cell adhesion to the vascular endothelium is a critical step of tumour metastasis. Endothelial surface molecule Thy-1 (CD90) is implicated in the metastatic process through its interactions with integrins and syndecans. However, how Thy-1 supports cell–cell adhesion in a dynamic mechanical environment is not known. Here we show that Thy-1 supports β 1 integrin- and syndecan-4 (Syn4)-mediated contractility-dependent mechanosignalling of melanoma cells. At the single-molecule level, Thy-1 is capable of independently binding α 5 β 1 integrin and syndecan-4 (Syn4) receptors. However, in the presence of both α 5 β 1 and Syn4, the two receptors bind cooperatively to Thy-1, to form a trimolecular complex. This trimolecular complex displays a unique phenomenon we coin ‘dynamic catch’, characterized by abrupt bond stiffening followed by the formation of catch bonds, where force prolongs the bond lifetime. Thus, we reveal a new class of trimolecular interactions where force strengthens the synergistic binding of two co-receptors and modulates downstream mechanosignalling. Cell adhesion molecules of the immunoglobulin superfamily bind cell surface receptors, such as integrins, on neighbouring cells, mediating cell–cell adhesion and transcellular communication [1] . Thy-1 (CD90) is a heavily N-glycosylated single v-type immunoglobulin (Ig) domain-containing glycoprotein, probably of primordial origin within the immunoglobulin superfamily [2] . It is linked to the outer leaflet of the plasma membrane via a carboxy-terminal glycophosphatidylinositol anchor, where it binds integrins in a variety of tissue-specific contexts, including α M β 2 (Mac-1) on leukocytes [3] , [4] , α v β 3 on melanoma cells [5] and neurons [6] , [7] , and α v β 5 on lung fibroblasts [8] . For a full review, see ref. 9 . Binding to α v integrins is mediated by Thy-1’s Arg-Leu-Asp (RLD) motif, as mutation to non-functional Arg-Leu-Glu abolishes binding [6] , [7] , [8] . Thy-1 also binds heparin sulphate proteoglycans (HSPGs), including syndecan-4 (Syn4), through a conserved polycationic motif in the C–C’ strand loop motif [7] , [10] . In patients with metastatic melanoma, Thy-1 is highly expressed on both the venous and lymphatic endothelium, where it facilitates metastasis in experimental models of melanoma [11] , [12] . Thy-1 expression is also enriched on human tumour-associated endothelium and lymphatic vessels [13] . This poses an important question as to whether endothelial expression of Thy-1 mediates binding and extravasation of circulating tumour cells responsible for secondary tumour site formation. However, the role of force on its interactions with receptors has not been explored. Integrins and syndecans are two primary receptor families that mediate adhesion, and their relative functional contributions to cell–extracellular matrix and cell–cell interactions remain under investigation. Growing evidence indicates that synergistic signalling is required for proper control of adhesive function and cell phenotype regulation in response to the external environment [14] , [15] . Specifically, Syn4 engagement of the HepII domain (type III repeats 12–14) of fibronectin (Fn) promotes intracellular signalling through protein kinase Cα (PKCα) and Rho family GTPases [15] , [16] , [17] , [18] . This, in concert with focal adhesion kinase (FAK), Src and other signalling modules controlled via integrin ligation, directs focal adhesion (FA) assembly and maturation [19] . Importantly, such assembly processes are regulated by mechanical force [20] , [21] , [22] . In particular, nascent complexes, including scaffolding molecules such as paxillin (Pxn), form at the leading edge, while myosin II-mediated tension leads to recruitment and activation of accessory proteins, promoting growth of the complex distal to the leading edge [23] . Increased mechanical tension leads to activation of downstream signalling molecules such as FAK and Rho family guanine nucleotide exchange factors (GEFs) [24] , [25] . Cells are able to sense the mechanical properties of their environment and alter their phenotype, giving rise to developmentally regulated and/or pathological processes [26] . However, the molecular mechanisms by which mechanical force is transduced into biochemical signals remains obscure [27] . Single-molecule approaches (that is, the biomembrane force probe (BFP)) have been extensively used to study force regulation of protein–protein interactions, determine protein conformational changes and understand signal initiation [28] , [29] , [30] , [31] , dissecting the relative contribution of individual proteins from complex molecular cohorts [32] . For example, single-molecule studies have elucidated the catch bond behaviour—bonds can be stabilized rather than disrupted by force [33] , [34] . Catch bonds are probably essential to key cell physiological events that occur in conditions where forces are externally applied or internally generated by the cell, such as adhesion enhancement of circulating cells and bacteria under shear stress or during receptor mechanosignalling [35] , [36] , [37] . They may also play fundamental roles in pathological progression, such as in the case of primary tumour metastasis. In this study, we investigate the adhesion of A375 human melanoma cells during cell contact of Thy-1-presenting surfaces, thus mimicking inflamed and/or tumour-associated endothelium. We describe a role for Thy-1 during myosin II-mediated adhesion maturation, and this response was critically dependent on integrin α 5 β 1 . We then use BFP to investigate the specific binding of Thy-1 to A375 cell receptors. In addition to the α 5 β 1 receptor, Thy-1 also interacts with a co-receptor, Syn4. Adhesion frequency analysis in the absence of force shows that the receptor and co-receptor bind cooperatively to form a trimolecular complex, synergistically increasing the number of bonds beyond the sum of Thy-1–α 5 β 1 and Thy-1–Syn4 bimolecular bonds. Surprisingly, we find a complex mechanical regulation of adhesive bonds at the single-molecule level: tensile force prolongs the bond lifetime (that is, catch bonds). In contrast to the well-known catch bonds of bimolecular systems, such as cell adhesion receptors (integrins [28] , [38] , [39] , selectins [40] , [41] , glycoprotein Ibα [30] , [42] , E-cadherin [43] and FimH [44] ), the T-cell receptor [31] and cytoskeletal linkages [45] , [46] , the Thy-1 catch bond is strongly correlated with a bond-stiffening phenotype, termed ‘dynamic catch’, which partially shifts force to the already engaged but unstretched co-receptor Syn4. Thus, the data reveal a unique, previously unreported class of receptor–ligand bonds whereby force tightens co-receptor engagement that is required for force-mediated adhesion signalling. Thy-1 enables β 1 integrin-mediated adhesion maturation It has recently been reported that Thy-1 mediates melanoma cell adhesion to the endothelium, facilitating tumour metastasis in the B16/F10 model [12] . This interaction is mainly attributed to integrin α v β 3 engagement; however, the downstream signalling responses and adhesive phenotype of cells engaging Thy-1 are less well known. We investigated adhesions formed during melanoma cell spreading on Thy-1, in comparison with the well-studied extracellular matrix ligand Fn. A375 human melanoma cells plated on Thy-1-presenting surfaces showed robust FA formation as indicated by immunostaining for Pxn and active FAK (FAK-pY397), including a spectrum of morphometric and biochemical characteristics similar to those observed on Fn and indicative of the adhesion maturation cycle ( Fig. 1a–c ). FAK activity was significantly elevated in adhesions >1 μm 2 and was positively correlated with adhesion size ( Fig. 1b,c ). As FAK is activated on tension, this provides a potential marker of force-mediated signalling [24] . Treatment with myosin II inhibitor, blebbistatin, disrupted adhesion maturation and promoted nascent adhesions on both Thy-1 and Fn substrates, indicating that myosin-generated forces on the adhesion complex are necessary for proper maturation and signalling ( Fig. 1b,c ). We also verified that de novo protein deposition on substrates (for example, cellular fibronectin assembly) was not effecting our measurements by treating cells with cycloheximide before spreading and adhesion analysis; cycloheximide (CHX) treatment did not affect FA assembly and FAK activation, nor did we detect deposited Fn on substrates ( Supplementary Fig. 1 ). As integrins are the main receptors required for fibronectin-dependent mechanotransduction [47] , we investigated which integrin receptors were responsible for A375 adhesion signalling on Thy-1 using function-blocking monoclonal antibodies (mAbs). When α v β 3 integrin was blocked, adhesion size-dependent FAK activity was largely unaffected and FAK signalling remained correlated with adhesion size, although overall adhesion size was slightly decreased ( Fig. 1b,c and Supplementary Fig. 2a ); this is consistent with a role for α v β 3 ligation of Thy-1 (ref. 48 ). In contrast, when β 1 integrin was blocked, FAK activity in large adhesions (>1 μm 2 ) was specifically decreased, and FAK activation as a function of adhesion size, and thus myosin II tension, was less well correlated ( Fig. 1b,c ). These data suggest that β 1 integrin, facilitates Thy-1-mediated adhesion signalling modulated by myosin II-dependent contractility. 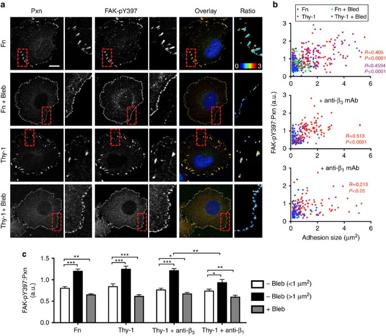Figure 1: Thy-1 mediates β1integrin and myosin II-dependent adhesion maturation in A375 cells. (a) Immunofluorescence images of Pxn, FAK-pY397, overlays (depicting Pxn in green and FAK-pY397 in red), and ratiometric quantification of FAK activation in A375 cells spread on Thy-1 or fibronectin (Fn) with or without 25 μM blebbistatin (Bleb) treatment. The corresponding magnified views are indicated with red rectangles. Ratiometric FAK-pY397:Pxn data gives spatial and morphometric quantification per FA. Expanded views on the right of each group correspond to the area indicated with red rectangles in the whole cell views on the left. The range of ratio values (in arbitrary values) is indicated by colour scale. Scale bar, 10 μm. (b) Distributions of FAK activation (FAK-pY397:Pxn) versus adhesion size for representative cells in the absence or presence of blebbistatin. β1and β1integrin blocking mAbs were incubated with A375 cells for 30 min in suspension before plating. Statistically significant Pearson’s correlation values and two-tailedP-values are indicated. (c) Mean±s.e.m. for non-treated adhesions binned into groupings <1 μm2, >1 μm2, or non-binned adhesions treated with Bleb. Data sets representn>800 adhesions from 9 cells or greater from each treatment condition. One representative of two independent experiments is shown. *P<0.05; **P<0.01; ***P<0.001; as assessed by unpaired, two-tailed Student’st-test. Figure 1: Thy-1 mediates β 1 integrin and myosin II-dependent adhesion maturation in A375 cells. ( a ) Immunofluorescence images of Pxn, FAK-pY397, overlays (depicting Pxn in green and FAK-pY397 in red), and ratiometric quantification of FAK activation in A375 cells spread on Thy-1 or fibronectin (Fn) with or without 25 μM blebbistatin (Bleb) treatment. The corresponding magnified views are indicated with red rectangles. Ratiometric FAK-pY397:Pxn data gives spatial and morphometric quantification per FA. Expanded views on the right of each group correspond to the area indicated with red rectangles in the whole cell views on the left. The range of ratio values (in arbitrary values) is indicated by colour scale. Scale bar, 10 μm. ( b ) Distributions of FAK activation (FAK-pY397:Pxn) versus adhesion size for representative cells in the absence or presence of blebbistatin. β 1 and β 1 integrin blocking mAbs were incubated with A375 cells for 30 min in suspension before plating. Statistically significant Pearson’s correlation values and two-tailed P -values are indicated. ( c ) Mean±s.e.m. for non-treated adhesions binned into groupings <1 μm 2 , >1 μm 2 , or non-binned adhesions treated with Bleb. Data sets represent n >800 adhesions from 9 cells or greater from each treatment condition. One representative of two independent experiments is shown. * P <0.05; ** P <0.01; *** P <0.001; as assessed by unpaired, two-tailed Student’s t -test. Full size image α 5 β 1 –Thy-1 catch bonds require cell surface presentation To verify that Thy-1 and α 5 β 1 integrin directly interact and to investigate potential force regulation of this interaction, we characterized the two-dimensional kinetics of single bonds between Thy-1 and a recombinant α 5 β 1 ectodomain (α 5 β 1 –Fc) or native α 5 β 1 expressed on a cell line (K562) using a BFP ( Fig. 2a ). The K562 cell model system was chosen due to its small repertoire of expressed integrins ( Supplementary Fig. 3a ) and HSPGs [49] , [50] , allowing precise control over interaction specificity. Bond lifetimes were measured by BFP force-clamp assay [51] , where the duration before bond dissociation is measured under different forces ( Fig. 3a ). The Thy-1–α 5 β 1 bond lifetime ‹ t α5β1-Fc ›, measured with purified α 5 β 1 ectodomain ( Fig. 2b , grey square) exhibited ordinary slip bond behaviour—bond lifetime decreases with increasing force. This is in contrast to the α 5 β 1 bond with fibronectin, which shows a catch bond—bond lifetime increases despite increasing force [38] . However, when α 5 β 1 –K562 cell bond lifetimes ‹ t K562 › were measured, a striking triphasic force dependence was observed ( Fig. 2b , black circle). A slip bond was observed in the regime <20 pN, a catch bond was observed from 20–35 pN and, after reaching a peak, a second slip bond was observed. Thus, a significant discrepancy exists between the force regulation of Thy-1 bonds on the K562 cell surface compared with the purified α 5 β 1 receptor. 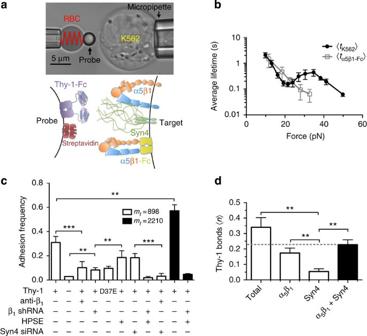Figure 2: Thy-1 forms catch bonds and binds cooperatively to a K562 cell. (a) Depiction of setup and interacting molecules. An RBC with a probe bead attached to apex (left) was aligned against a target K562 cell (right). The molecules of interest: α5β1and Syn4 were expressed on a target K562 cell or recombinant α5β1was coated on a target bead, and Thy-1 was coated on the probe bead. (b) Force regulation of bond lifetime of Thy-1 versus receptor-bearing targets. Bond lifetime (mean±s.e.m.) of Thy-1–K562 (black circle) and Thy-1–α5β1-Fc (grey square) bonds is plotted versus force. (c) Binding specificity. Adhesion frequencies between beads (coated with and without Thy-1 or D37E mutant) and K562 cells (with and without α5β1or Syn4 knockdown; or HPSE treatment) in the absence and presence of 20 μg ml−1anti-β1mAb (AIIB2). Measurements at surface densities of 898 and 2,210 μm−2are denoted by the white and black bars, respectively. The treatment combinations for each experiment are indicated. Data are presented as mean±s.e.m. of 3–5 pairs of cells and beads repeatedly contacting 50 times with fixed 0.5-s contact duration. *P<0.05; **P<0.01; ***=P<0.001, as assessed by unpaired, two-tailed Student’st-test. (d) The average bond numbers ‹n› derived from adhesion frequencyPa(same data fromc) by equation 1 (see Methods) for bimolecular bond (Thy-1–α5β1or Thy-1–Syn4) and trimolecular bond (Thy-1–α5β1+Syn4). The reference (grey) line depicts the ‹nα5β1›+‹nSyn4› value (black bar). Figure 2: Thy-1 forms catch bonds and binds cooperatively to a K562 cell. ( a ) Depiction of setup and interacting molecules. An RBC with a probe bead attached to apex (left) was aligned against a target K562 cell (right). The molecules of interest: α 5 β 1 and Syn4 were expressed on a target K562 cell or recombinant α 5 β 1 was coated on a target bead, and Thy-1 was coated on the probe bead. ( b ) Force regulation of bond lifetime of Thy-1 versus receptor-bearing targets. Bond lifetime (mean±s.e.m.) of Thy-1–K562 (black circle) and Thy-1–α 5 β 1 -Fc (grey square) bonds is plotted versus force. ( c ) Binding specificity. Adhesion frequencies between beads (coated with and without Thy-1 or D37E mutant) and K562 cells (with and without α 5 β 1 or Syn4 knockdown; or HPSE treatment) in the absence and presence of 20 μg ml −1 anti-β 1 mAb (AIIB2). Measurements at surface densities of 898 and 2,210 μm −2 are denoted by the white and black bars, respectively. The treatment combinations for each experiment are indicated. Data are presented as mean±s.e.m. of 3–5 pairs of cells and beads repeatedly contacting 50 times with fixed 0.5-s contact duration. * P <0.05; ** P <0.01; ***= P <0.001, as assessed by unpaired, two-tailed Student’s t -test. ( d ) The average bond numbers ‹ n › derived from adhesion frequency P a (same data from c ) by equation 1 (see Methods) for bimolecular bond (Thy-1–α 5 β 1 or Thy-1–Syn4) and trimolecular bond (Thy-1–α 5 β 1 +Syn4). The reference (grey) line depicts the ‹ n α5β1 ›+‹ n Syn4 › value (black bar). 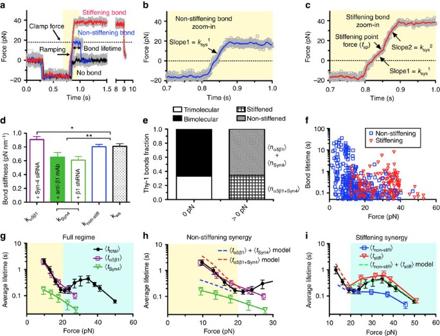Figure 3: Trimolecular bonds exhibit ‘Dynamic catch’ behaviour. (a) Representative force versus time overlapping plots showing no bond (black), non-stiffening bond (blue) and stiffening bond (red) events. Data (points, grey) were acquired at 1,200 fps and were smoothed using the Savitzky–Golay method. (b,c) Representative force versus time zoom-in plots in the ramping phase showing non-stiffening (b) and stiffening (c) signatures. The force at SP (fsp), the stiffness before SP (ksys1) and after SP (ksys2) are indicated. Zero forces are shown by dotted lines. (d) Mean±s.e.m. (of >50 measurements) stiffness of Thy-1–K562 molecular complexes measured by BFP, from left to right:kα5β1obtained by Syn4 siRNA treatment,kSyn4obtained by anti-β1 mAb and β1 shRNA treatment, respectively,knon-stifffor all non-stiffening bonds andkwscalculated as the ‹n› weighted sum ofkα5β1andkSyn4. *P<0.05; **P<0.01 as assessed by unpaired, two-tailed Student’st-test. (e) The relative fraction of Thy-1 bonds: the left column shows trimolecular (empty) versus bimolecular (solid) bond compositions at zero force; the right column shows stiffened (grid) versus non-stiffened (shaded) bond compositions at non-zero force in the ramping phase. (f) Scatter plots of bond lifetimes versus corresponding clamp forces. Individual lifetimes (scatter points) fromawere colour-coded for non-stiffening (blue) and stiffening (red) bonds, respectively. (g) Plots of lifetime (mean±s.e.m.) versus force of Thy-1–α5β1(‹tα5β1›, Syn4 siRNA treated, purple square), Thy-1–Syn4 (‹tSyn4›, β1shRNA treated, green triangle) bimolecular bonds and total Thy-1–K562 bonds (‹ttotal›, untreated, black circle) for the full force regime investigated. (h) Non-stiffening synergy zoom-in. The low force regime fromg(yellow) is highlighted. Weighted sum (by respective ‹n› inFig. 2d) of bimolecular bonds (‹tα5β1›+‹tSyn4›, blue dashed line) and calculated trimolecular bonds (‹tα5β1+Syn4›, red dashed line) are shown. (i) Stiffening synergy zoom-in. The high force regime fromg(turquoise) is highlighted. Non-stiffening bonds ((‹tnon-stiff›+‹tstiff›, green dashed line, ‹tnon-stiff›, blue square), stiffening bonds (‹tstiff›, red triangle) and their weighted sum (by respective ‹n› in corresponding force regime) are shown in the high force regime. Full size image Figure 3: Trimolecular bonds exhibit ‘Dynamic catch’ behaviour. ( a ) Representative force versus time overlapping plots showing no bond (black), non-stiffening bond (blue) and stiffening bond (red) events. Data (points, grey) were acquired at 1,200 fps and were smoothed using the Savitzky–Golay method. ( b , c ) Representative force versus time zoom-in plots in the ramping phase showing non-stiffening ( b ) and stiffening ( c ) signatures. The force at SP ( f sp ), the stiffness before SP ( k sys 1 ) and after SP ( k sys 2 ) are indicated. Zero forces are shown by dotted lines. ( d ) Mean±s.e.m. (of >50 measurements) stiffness of Thy-1–K562 molecular complexes measured by BFP, from left to right: k α5β1 obtained by Syn4 siRNA treatment, k Syn4 obtained by anti-β1 mAb and β1 shRNA treatment, respectively, k non-stiff for all non-stiffening bonds and k ws calculated as the ‹ n › weighted sum of k α5β1 and k Syn4 . * P <0.05; ** P <0.01 as assessed by unpaired, two-tailed Student’s t -test. ( e ) The relative fraction of Thy-1 bonds: the left column shows trimolecular (empty) versus bimolecular (solid) bond compositions at zero force; the right column shows stiffened (grid) versus non-stiffened (shaded) bond compositions at non-zero force in the ramping phase. ( f ) Scatter plots of bond lifetimes versus corresponding clamp forces. Individual lifetimes (scatter points) from a were colour-coded for non-stiffening (blue) and stiffening (red) bonds, respectively. ( g ) Plots of lifetime (mean±s.e.m.) versus force of Thy-1–α 5 β 1 (‹ t α5β1 ›, Syn4 siRNA treated, purple square), Thy-1–Syn4 (‹ t Syn4 ›, β 1 shRNA treated, green triangle) bimolecular bonds and total Thy-1–K562 bonds (‹ t total ›, untreated, black circle) for the full force regime investigated. ( h ) Non-stiffening synergy zoom-in. The low force regime from g (yellow) is highlighted. Weighted sum (by respective ‹ n › in Fig. 2d ) of bimolecular bonds (‹ t α5β1 ›+‹ t Syn4 ›, blue dashed line) and calculated trimolecular bonds (‹ t α5β1+Syn4 ›, red dashed line) are shown. ( i ) Stiffening synergy zoom-in. The high force regime from g (turquoise) is highlighted. Non-stiffening bonds ((‹ t non-stiff ›+‹ t stiff ›, green dashed line, ‹ t non-stiff ›, blue square), stiffening bonds (‹ t stiff ›, red triangle) and their weighted sum (by respective ‹ n › in corresponding force regime) are shown in the high force regime. Full size image α 5 β 1 , Syn-4 and Thy-1 cooperatively form a trimolecular complex To investigate potential alternate interactions with the K562 cell compared with the purified system, we used an adhesion frequency assay to measure binding specificity. As previously reported [51] , the absence ( Fig. 3a , black trace) or presence ( Fig. 3a , blue and red traces) of a bond is detected by the presence of a tensile force upon K562 cell retraction from the Thy-1 BFP, allowing calculation of adhesion frequency from repeated touches ( Fig. 2c ). To verify binding specificity, we measured K562 cell binding to a probe not coated with Thy-1, which reduced adhesion frequency to a nonspecific level. Blocking with an anti-β 1 ( Fig. 2c ) or an anti-α 5 ( Supplementary Fig. 4 ) mAb decreased adhesion frequency by threefold, as did stable knockdown of β 1 expression using RNA interference (RNAi), but neither abolished adhesion completely ( Fig. 2c ). Mutation of Thy-1 (D37E) in the purported integrin-binding motif, RLD, suppressed the binding to a similar degree as β 1 and α 5 antibody blockade did, confirming this as the binding motif for α 5 β 1 . As α 5 β 1 is the only constitutively expressed RGD-binding integrin on the K562 cells used [49] ( Supplementary Fig. 3a ), this data indicates that the binding events were primarily mediated by Thy-1–α 5 β 1 interactions. Incomplete blocking by anti-β 1 or anti-α 5 mAbs suggested an additional adhesive interaction between the cell surface and Thy-1 ( Fig. 2d and Supplementary Fig. 3 ). It was reported that Thy-1 contains a putative polycationic heparin-binding sequence, which mediates binding to the HSPG, Syn4, and activation of PKCα [7] . When K562 cells were pretreated with heparinase (HPSE) to cleave heparin sulphate glycosaminoglycans (GAGs) from the cell surface, adhesions were reduced; Syn4 knockdown by small interfering RNA (siRNA) showed similar reduction ( Fig. 2c ). Dual inhibition of both α 5 β 1 and Syn4 (with combined treatments of β 1 knockdown+HPSE, anti-β 1 mAb+Syn4 knockdown or anti-α 5 mAb+HPSE) abrogated the total Thy-1–K562 adhesions to the level of nonspecific binding ( Fig. 2c and Supplementary Fig. 4 ). The same inhibition results were obtained with a higher Thy-1 coating density ( Fig. 2c , solid bars). These results suggested that HSPGs, in particular Syn4, is a co-receptor for Thy-1 ( Fig. 2c , solid bars). As the respective binding sites for α 5 β 1 and Syn4 on Thy-1 are distinct [52] , the K562 cell may adhere to the Thy-1 probe via a bimolecular bond (Thy-1–α 5 β 1 or Thy-1–Syn4) and/or a trimolecular bond (Thy-1–α 5 β 1 +Syn4), or their combinations. To determine the bond composition, we calculated the average numbers of Thy-1–α 5 β 1 or Thy-1–Syn4 bimolecular bonds (‹ n α5β1 › or ‹ n Syn4 ›) from the respective adhesion frequencies measured when Syn4 or α 5 β 1 was knocked down, respectively, and compared their sum with the average number of total bonds (‹ n total ›) from the adhesion frequency measured with no treatments (Methods, equation (1)) [53] . Remarkably, the sum of the two bimolecular bond average numbers, ‹ n α5β1 ›=0.173±0.032 and ‹ n Syn4 ›=0.054±0.018, was only 0.227±0.032, significantly smaller than the average number of total bonds, ‹ n total ›=0.341±0.062 ( Fig. 2d , P <0.01). We used flow cytometry to verify that β 1 or Syn4 knockdown did not affect the expression of the alternate receptor ( Supplementary Fig. 3c ). These results indicate that the Thy-1 trimolecular bond accounts for the remaining portion: ‹ n α5β1+Syn4 ›=‹ n total ›−(‹ n α5β1 ›+‹ n Syn4 ›) (Methods, equation (2)). These results also demonstrate that Syn4 and α 5 β 1 bind cooperatively to exert a synergistic effect on complex formation, as ‹ n total › is greater than ‹ n α5β1 ›+‹ n Syn4 ›, thus forming a greater number of total bonds than the sum of bonds formed by these two receptors independently [54] . This calculation assumes that the respective Thy-1 bonds with α 5 β 1 and Syn4 measured when the other receptor was knocked down (that is, bimolecular bonds with only a single receptor species present) remain the same as when both receptors are expressed. Note that relaxing this assumption only changes the type of synergy observed, but not the amount. Should the bimolecular bonds for one receptor decrease in the presence of the other receptor (that is, inhibition or negative cooperativity), then either the alternate receptor’s bimolecular bonds or the trimolecular bonds or both must increase (that is, synergy or positive cooperativity) to account for the total number of bonds observed. Thy-1 supports a unique bond stiffening phenotype As a deterministic property of a molecular complex, stiffness has been used to identify the type of selectins [55] and the conformation of integrin [29] . We therefore measured the stiffness of the Thy-1–α 5 β 1 and Thy-1–Syn4 bimolecular bonds and compared them with the total bonds that might also contain Thy-1–α 5 β 1 +Syn4 trimolecular bonds. The molecular bond stiffness was derived from the force-extension data (see Fig. 4a ) from the ramping phase during the BFP retraction ( Fig. 3a ) [29] , [55] . The model consisted of a set of springs to distinguish contributions from various elements to the different slopes observed during force loading (see Fig. 4c and Methods). The Thy-1–Syn4 bond stiffness, measured under β 1 short hairpin RNA (shRNA) or anti-β 1 mAb treatment, had similar values of k Syn4 =0.610±0.053 or 0.653±0.067 pN nm −1 , respectively ( Fig. 3d ). The Thy-1–α 5 β 1 bond stiffness, measured under Syn4 siRNA treatment, was stiffer, k α5β1 =0.908±0.045 pN nm −1 . When the ramping phase of the force–time curves were interrogated further, we unexpectedly identified two types of bonds with distinct molecular elasticity signatures: (1) non-stiffening bonds, featuring a single linear segment in the force-ramping phase ( Fig. 3b ) and (2) stiffening bonds, featuring an abrupt kink (denoted stiffening point, SP) that separated the ramping phase into two linear segments, the second having a significantly steeper slope ( Fig. 3c ). The stiffness of the non-stiffening bond was k non-stiff =0.804±0.033 pN nm −1 . This value is between those of the Thy-1–α 5 β 1 and Thy-1–Syn4 bimolecular bonds ( Figs 3d and 4b ), but equivalent to the weighted sum of the stiffness of Thy-1–α 5 β 1 and Thy-1–Syn4 bonds, k WS =(‹ n α5β1 › k α5β1 +‹ n Syn4 › k Syn4 )/(‹ n α5β1 ›+‹ n Syn4 ›)=0.811±0.037 pN nm −1 ( Fig. 3d ). 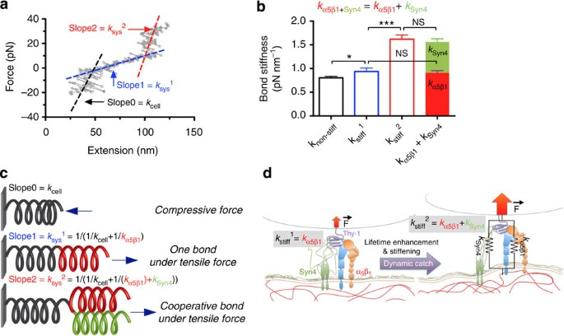Figure 4: Biophysical mechanism of the dynamic catch. (a) Measurement of molecular stiffness by BFP; a representative extension versus force plot showing the first kink in the force-ramping phase at ~0 pN. The slope of the linear fit to the compressive loading segment (slope0 of the black dashed line) equals the stiffnesskcellof a cellular spring. The slope of the linear fit to the tensile loading segment (slope1 of the blue dashed line) equals the stiffness of a systemksysthat consists of the cellular spring and the molecular spring in series. The system stiffness before (ksys1) and after (ksys2) SP are calculated from respective tensile loading segments (slope1 of the blue dashed line and slope2 of the red dashed line) the same way as the non-stiffening bonds. (b) Stiffness (mean±s.e.m. of >50 measurements) of Thy-1–K562 molecular complexes, left to right:knon-stifffor non-stiffening bonds;kstiff1(=ksys1) before SP for stiffening bonds;kstiff2(=1/(1/ksys2−1/kcell)) after SP for stiffening bonds;kα5β1+kSyn4, sum ofknon-stiffobtained with Syn4 and β1knockdown K562 cells. NS, not significant, *P<0.05; **P<0.01; ***P<0.001, as assessed by unpaired, two-tailed Student’st-test. (c) Mechanical model of the trimolecular system corresponding toa.kα5β1andkSyn4are the bimolecular stiffness for Thy-1–α5β1and Thy-1–Syn4, respectively.kα5β1+Syn4=kα5β1+kSyn4is the trimolecular stiffness for Thy-1–α5β1+Syn4. (d) A model for Thy-1–α5β1+Syn4 dual-receptor engagement and dynamic catch. A trimolecular complex exhibiting synergistic binding is formed during initial contact of Thy-1 and the α5β1+Syn4-bearing cell. When tensile force is applied to the complex, the interaction is strengthened (that is, catch bond formation) and stiffened, as Syn4 contributes to the molecular rigidity of the complex. The stiffness of the trimolecular complex is equivalent to the sum of the two bimolecular bonds (Thy-1–α5β1or Thy-1–Syn4) in parallel. Figure 4: Biophysical mechanism of the dynamic catch. ( a ) Measurement of molecular stiffness by BFP; a representative extension versus force plot showing the first kink in the force-ramping phase at ~0 pN. The slope of the linear fit to the compressive loading segment (slope0 of the black dashed line) equals the stiffness k cell of a cellular spring. The slope of the linear fit to the tensile loading segment (slope1 of the blue dashed line) equals the stiffness of a system k sys that consists of the cellular spring and the molecular spring in series. The system stiffness before ( k sys 1 ) and after ( k sys 2 ) SP are calculated from respective tensile loading segments (slope1 of the blue dashed line and slope2 of the red dashed line) the same way as the non-stiffening bonds. ( b ) Stiffness (mean±s.e.m. of >50 measurements) of Thy-1–K562 molecular complexes, left to right: k non-stiff for non-stiffening bonds; k stiff 1 (= k sys 1 ) before SP for stiffening bonds; k stiff 2 (=1/(1/ k sys 2 −1/ k cell )) after SP for stiffening bonds; k α5β1 + k Syn4 , sum of k non-stiff obtained with Syn4 and β 1 knockdown K562 cells. NS, not significant, * P <0.05; ** P <0.01; *** P <0.001, as assessed by unpaired, two-tailed Student’s t -test. ( c ) Mechanical model of the trimolecular system corresponding to a . k α5β1 and k Syn4 are the bimolecular stiffness for Thy-1–α 5 β 1 and Thy-1–Syn4, respectively. k α5β1+Syn4 = k α5β1 + k Syn4 is the trimolecular stiffness for Thy-1–α 5 β 1 +Syn4. ( d ) A model for Thy-1–α 5 β 1 +Syn4 dual-receptor engagement and dynamic catch. A trimolecular complex exhibiting synergistic binding is formed during initial contact of Thy-1 and the α 5 β 1 +Syn4-bearing cell. When tensile force is applied to the complex, the interaction is strengthened (that is, catch bond formation) and stiffened, as Syn4 contributes to the molecular rigidity of the complex. The stiffness of the trimolecular complex is equivalent to the sum of the two bimolecular bonds (Thy-1–α 5 β 1 or Thy-1–Syn4) in parallel. Full size image To further confirm our hypothesis that non-stiffening bonds consist of two species, we interrogated the frequency distribution of Thy-1–K562 non-stiffening bonds. In non-treated cells, the bond stiffness histogram was fit with a bimodal distribution with peaks at 0.63 and 0.96 pN nm −1 , in excellent agreement with the measured values for Thy-1–Syn4 and Thy-1–α 5 β 1 , respectively ( Supplementary Fig. 5a ). To directly relate the subpopulation of higher stiffness (~0.9 pN nm −1 ) from our analysis to the Thy-1–α 5 β 1 bond, we measured the bond stiffness with recombinant α 5 β 1 -Fc. We found that the bond stiffness of Thy-1–K562 with Syn4 knockdown is comparable to that of α 5 β 1 -Fc in terms of absolute values ( Supplementary Fig. 5b ) and distribution ( Supplementary Fig. 5c ), suggesting that the non-stiffening bonds predominately consisted of Thy-1–α 5 β 1 and Thy-1–Syn4 bimolecular bonds. Supporting this hypothesis, the prevalence of stiffening events was 0.34 (over total bond events, Fig. 3e ), comparable to the fraction of trimolecular bonds, 0.33, calculated from the adhesion frequency analysis (see Methods). Addition of the function-blocking anti-β 1 mAb completely eliminated the stiffening phenomenon ( Fig. 5b ), supporting the hypothesis that these represented predominately the Thy-1–α 5 β 1 +Syn4 trimolecular bonds. 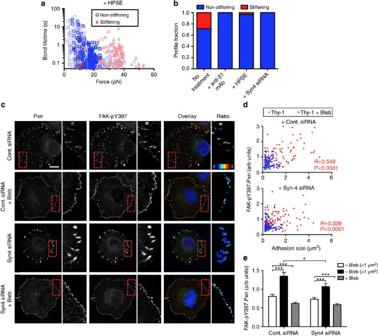Figure 5: Syn4 engagement is required for dynamic catch and contractility-dependent adhesion maturation. (a) Scatter plot of bond lifetime versus clamp force for HPSE-treated K562 cells. The measurements and colour codes are the same as the data ofFig. 3f, which are overlaid with the same but dimmed colours for comparison. (b) Fraction of non-stiffening (blue) versus stiffening (red) Thy-1–K562 bonds at the absence and presence of anti-β1mAb, HPSE and those with Syn4 siRNA in K562 cells. The same treatment conditions were used asFig. 2c. (c) Immunofluorescence images of Pxn, FAK-pY397, overlays (depicting Pxn in green and FAK-pY397 in red), and ratiometric quantification of FAK activation in A375 cells spread on Thy-1 with control (Cont.) or Syn4 siRNA, and with or without 25 μM blebbistatin. Expanded views correspond to the area indicated with a red rectangle. The range of ratio values (in arbitrary values) is indicated by colour scale. Scale bar, 10 μm. (d) Distributions of FAK activation (FAK-pY397:Pxn) versus adhesion size for individual adhesions of representative Cont. (upper) or Syn4 siRNA-treated (lower) cells with or without 25 μM blebbistatin. Statistically significant Pearson’s correlation values and two-tailedP-values are indicated. (e) Mean±s.e.m. for non-treated adhesions binned into groupings <1 μm2, >1 μm2, or non-binned adhesions treated with Bleb. Data sets representn>800 adhesions from ten cells or greater for each treatment condition. One representative of two independent experiments is shown. *P<0.05; **P<0.01; ***P<0.001; as assessed by unpaired, two-tailed Student’st-test. Figure 5: Syn4 engagement is required for dynamic catch and contractility-dependent adhesion maturation. ( a ) Scatter plot of bond lifetime versus clamp force for HPSE-treated K562 cells. The measurements and colour codes are the same as the data of Fig. 3f , which are overlaid with the same but dimmed colours for comparison. ( b ) Fraction of non-stiffening (blue) versus stiffening (red) Thy-1–K562 bonds at the absence and presence of anti-β 1 mAb, HPSE and those with Syn4 siRNA in K562 cells. The same treatment conditions were used as Fig. 2c . ( c ) Immunofluorescence images of Pxn, FAK-pY397, overlays (depicting Pxn in green and FAK-pY397 in red), and ratiometric quantification of FAK activation in A375 cells spread on Thy-1 with control (Cont.) or Syn4 siRNA, and with or without 25 μM blebbistatin. Expanded views correspond to the area indicated with a red rectangle. The range of ratio values (in arbitrary values) is indicated by colour scale. Scale bar, 10 μm. ( d ) Distributions of FAK activation (FAK-pY397:Pxn) versus adhesion size for individual adhesions of representative Cont. (upper) or Syn4 siRNA-treated (lower) cells with or without 25 μM blebbistatin. Statistically significant Pearson’s correlation values and two-tailed P -values are indicated. ( e ) Mean±s.e.m. for non-treated adhesions binned into groupings <1 μm 2 , >1 μm 2 , or non-binned adhesions treated with Bleb. Data sets represent n >800 adhesions from ten cells or greater for each treatment condition. One representative of two independent experiments is shown. * P <0.05; ** P <0.01; *** P <0.001; as assessed by unpaired, two-tailed Student’s t -test. Full size image α 5 β 1 and Syn4 cooperate to form catch bonds with Thy-1 We next analysed the mechanical regulation of Thy-1–α 5 β 1 and Thy-1–Syn4 bimolecular bonds on the K562 cell surface, as well as the total bonds that might contain the Thy-1–α 5 β 1 +Syn4 trimolecular complex. As demonstrated with purified α 5 β 1 ectodomain ( Fig. 2b ), the Thy-1–α 5 β 1 bond lifetime ‹ t α5β1 ›, measured with Syn4 siRNA- or HPSE-treated K562 cells ( Fig. 3g , purple, and Supplementary Fig. 6a,c ), exhibited a slip bond. The Thy-1–Syn4 bond lifetime ‹ t Syn4 ›, measured under β 1 shRNA or anti-β 1 mAb treatment, also exhibited ordinary slip bond behaviour ( Fig. 3g , green, and Supplementary Fig. 6b,d ). Given that total K562 bonds ‹ t total › exhibited catch bonds in the regime of 20–35 pN ( Fig. 2b ), this is surprising because the addition of two slip bonds should not result in a catch bond or an enhanced force resistance from 25 to 50 pN ( Fig. 3g , black). Moreover, the total bond lifetime was longer than the weighted sum of the two bimolecular bond lifetimes in the slip-bond regime of <20 pN (‹ t α5β1 ›+‹ t Syn4 › model, Fig. 3h ), indicating that the trimolecular bond lifetime accounts for the discrepancy. The trimolecular bond lifetime ‹ t α5β1+Syn4 ›, calculated by subtracting the lifetime contributions of the two bimolecular bonds from the total bond lifetime (Methods, equation (3)), was 78%, 10-fold and 53% longer than the Thy-1–α 5 β 1 , Thy-1–Syn4 and total (Thy-1–K562) bond lifetimes on average between 0–20 pN, respectively ( Fig. 3h ). These results demonstrate that the synergy between α 5 β 1 and Syn4 created a new type of bond, which not only increased the propensity of bond formation but also the prolonged bond lifetime. More importantly, it exhibited a qualitatively distinct response to mechanical force. Correlative stiffness and lifetime identifies dynamic catch To further test our hypothesis, we colour-coded individual events based on the presence and absence of bond stiffening during force ramping. When bond lifetimes were plotted versus force in a scattergram, an intriguing discrimination between the two populations emerged ( Fig. 3f ). The non-stiffening events distributed over the entire force range, while stiffening events only occurred at the force regime of >15 pN ( Fig. 3f ). Moreover, the stiffening events consistently demonstrated long lifetimes and mostly clustered in the force regime of 20–40 pN, overlapping the catch-bond regime ( Fig. 3f ). Segregating the lifetimes (all data; Fig. 3g,i , black circle) for each population reveals that the non-stiffening bond lifetimes ‹ t non-stiff › ( Fig. 3i , blue square) are responsible for the first slip-bond regime, while the stiffening bond lifetimes ‹ t stiff › ( Fig. 3i , red triangle) are primarily responsible for the catch-bond regime. The catch bond in the high force regime was solely attributed to the stiffening events. Furthermore, the total bond lifetime ‹ t total › can be approximated by the weighted sum of non-stiffening and stiffening bonds (‹ t non-stiff ›+‹ t stiff › model, Fig. 3i ). We term this novel phenomenon ‘dynamic catch’, as the molecular bond is both stiffened and its lifetime increased in response to an applied force over the sub-second timescale. More interestingly, the bimolecular (‹ t α5β1 ›+‹ t Syn4 › model, Fig. 3h ) and trimolecular (‹ t α5β1+Syn4 › model, Fig. 3h ) bond lifetimes measured in the force regime below the threshold for dynamic catch (<20 pN) fell into the extensions of the non-stiffening ( Fig. 3i , blue lines) and stiffening ( Fig. 3i , red lines) lifetimes, respectively, in the force regime above the threshold for dynamic catch (>20 pN). These lifetime trend consistencies ( Fig. 3i ) were confirmed by the bond fractions ( Fig. 3e ), suggesting that the dynamic catch uniquely corresponds to a Thy-1–α 5 β 1 +Syn4 trimolecular bond, while Thy-1–α 5 β 1 and Thy-1–Syn4 bimolecular bonds can only exhibit the non-stiffening bond phenotypes. Furthermore, the anchoring rupture force of glycophosphatidylinositol-anchored Thy-1 within the plasma membrane was measured as 30–50 pN ( Supplementary Fig. 6 ), within the range of forces tested in force-clamp assay. Syn4 is needed for dynamic catch and mature FAs Further supporting our hypothesis, we found that treatments of HPSE or Syn4 RNAi almost entirely eliminated the stiffening bond phenotype ( Fig. 5a,b ) and reduced the force required to rupture the bond ( Supplementary Fig. 7d ). In addition, force was no longer able to prolong the Thy-1–K562 bond lifetime with these treatments, and therefore the dynamic catch was completely abrogated ( Fig. 3g and Supplementary Fig. 5b,d ). These data demonstrate that co-receptor engagement is required for the dynamic catch and that co-receptor Syn4 engagement could be visualized with the BFP via the stiffening in the bond-loading profile. To investigate whether Syn4 additionally modulates integrin signalling during melanoma cell adhesion, we monitored contractility-dependent adhesion maturation with the Syn4 knockdown cells ( Fig. 5c ). Syn4 knockdown decreased FAK activation, most significantly in adhesions >1 μm 2 , although a positive correlation between FAK activation and adhesion size remained ( Fig. 5d,e ). Syn4 blocking also eliminated adhesions of larger size ( Fig. 5d ) and resulted in lower overall adhesion size ( Supplementary Fig. 2b ). Blebbistatin-treated adhesions remained similar in FAK activities and adhesion sizes comparing control and Syn4 siRNA-treated cells ( Fig. 5d,e and Supplementary Fig. 2b ). These data suggest that Syn4 engagement of Thy-1 is critical for adhesive signalling during myosin II-mediated adhesion maturation. Biophysical mechanism of the dynamic catch The abrupt slope change (that is, stiffness increase) of the stiffening bonds during force loading corresponds to a sudden strengthening of the Thy-1–α 5 β 1 +Syn4 trimolecular bonds that give rise to the dynamic catch ( Fig. 3f,i ). A comparison of the bond stiffness before ( k stiff 1 ) and after ( k stiff 2 ) the SP demonstrates that the stiffness of these bonds increases nearly 60%. Interestingly, the amount of sudden stiffness increase agrees with the value of bimolecular Thy-1–Syn4 bond stiffness ( k stiff 2 − k stiff 1 = k Syn4 , Fig. 4b ). These results can be explained by a two-state model of sequential loading of the α 5 β 1 and Syn4 legs in the trimolecular complex ( Fig. 4c ). The initial bond stiffness of the trimolecular bond is not significantly different than that of the bimolecular Thy-1–α 5 β 1 bond ( k stiff 1 = k α5β1 , Fig. 4b ). This suggests that the α 5 β 1 leg of the Thy-1–α 5 β 1 +Syn4 trimolecular bond bears the majority of the initial load in the first state ( Fig. 4c , middle panel). As force increases to the SP, the Syn4 leg may suddenly be tightened and contribute its full stiffness to the trimolecular bond in the second state, giving rise to the dynamic catch ( k stiff 2 = k α5β1+Syn4 = k α5β1 + k Syn4 , Fig. 4c , bottom panel). Interestingly, this suggests a potential force threshold may exist for the dynamic catch: with the distribution of SP forces, we observed that the force level was largely conserved at ~15 pN ( Supplementary Fig. 8a ). It has previously been demonstrated that Syn4 signalling can also modulate adhesion strength to Fn by regulating integrin internalization [56] and recycling [57] . Is the ‘dynamic catch’ a consequence of the biophysical properties of the Thy-1, α5β1 and Syn4 extracellular domains, or does rapid receptor signalling also contribute to the observed stiffening effect? To examine the potential contribution of Syn4 signalling, we performed the BFP experiments in the presence of inhibitors against dynamin (MiTMAB) to block dynamin-dependent integrin internalization or against Src (PP2) to block Syn4-dependent integrin recycling. Neither of these treatments had effects on the dynamic catch bond phenomenon observed ( Supplementary Fig. 8b,c ), suggesting that Syn4 signalling is not critical for this process. Considering all the data collected, we propose a model to describe the Thy-1–α 5 β 1 +Syn4 synergy ( Fig. 4d ): Syn4 cannot share mechanical force until the soft and highly flexible GAG chains are fully extended by the threshold force, at which point conformational changes in the integrin and/or ligand molecules may be elicited to yield the long-lived bond state. A possible explanation for the force threshold is that force deforms the axis of integrin, ligand and membrane/cortex to a certain degree, after which force can be transmitted to and shared by syndecan (that is, variable receptor length). Based on prior studies demonstrating that Thy-1 expression on the vascular endothelium (1) is enhanced by tumour-promoting inflammatory cytokines, (2) is specifically elevated in the tumour-associated endothelium and (3) plays a functional role in metastasis of melanoma in experimental models, we sought to investigate specific adhesive and mechanotransductive characteristics of melanoma cells to Thy-1-presenting surfaces. Extending from the extensively studied interaction between Thy-1 and α v β 3 integrin, we discovered α 5 β 1 integrin as a novel Thy-1 receptor mediating adhesion maturation on Thy-1 ( Fig. 1 ). At the single-molecule level, the Thy-1–α 5 β 1 interaction shows distinct phenomena: (1) it cooperates with Syn4 to increase bond formation ( Fig. 2d ); (2) force prolongs bond lifetime by converting the slip-bond behaviour of two individual bimolecular interactions to a catch bond of the trimolecular interaction ( Fig. 3g ); and (3) long-lived bond events reveal a stiffening signature in the force-loading phase ( Figs 3c and 4a ). These observations have not ever been reported in any single-molecule receptor–ligand studies. The intimate link between the last two phenomena demonstrates what we coin a ‘dynamic catch’, which is responsible for all Thy-1 catch bonds ( Fig. 3e–i ). Unlike previously described catch bond or cooperative binding co-factors [33] , [58] , such as allosteric regulation by neighbouring protein domains (that is, within the molecule) or soluble co-factors, our finding is distinct: the co-factor is a nearby co-receptor but not covalently associated with the first. Importantly, as circulating tumour cells are exposed to a complex haemodynamic environment during the their transit through the vasculature [59] , forces applied to non-covalent interactions between adhesion receptors are important perturbations that may regulate bond affinities and subsequent signalling. In the case of circulating tumour cells adhering to the endothelium during extravasation and eventual assembly of secondary tumour sites, dynamic catch bonds may facilitate tighter binding or survival signalling under shear stress at the vessel wall or during transcellular movement across the endothelial layer. Intriguingly, if the trimolecular complex is not allowed to form (that is, knockdown of Syn4), thereby also inhibiting dynamic catch, myosin II-mediated mechanosignalling through FAK is perturbed. This suggests that mechanotransductive events at the initial receptor–ligand complex level could lead to downstream mechanosignalling modulation within FAs. This is distinct from models of mechanotransduction/signalling involving conformational changes in stress-bearing cytoplasmic proteins, such as the cryptic exposure of vinculin-binding motifs within a mechanically stretched talin or exposure of Src-binding motifs within p130Cas [60] , [61] . Within the FA complex, a multitude of proteins, binding interactions and complex architecture make resolving mechanosignalling mechanisms at the molecular level a challenge. Here we show that force-induced binding changes occur at the cell surface, resulting in strengthening of a trimolecular complex under force, and alterations in mechanosignalling at the FA level strongly correlate to bond phenotypes at the single-molecule level. Alternative methods to determine trimolecular interactions, including immunoprecipitation or surface plasmon resonance (SPR), could be used; however, we stress that only by using single-molecule-sensitive force probes such as BFP were we able to measure the force responsiveness and dynamics of the complex, which were otherwise inaccessible using traditional methods. Intriguingly, biochemical signalling does not appear to be required for the formation of dynamic catch bonds. Syn4 was recently shown to act as a hair trigger leading to integrin internalization via downstream activation of a PKCα-RhoG signalling axis and dynamin-dependent scission of endocytic vesicles [56] . When dynamin was inhibited, no change in the dynamic catch bond phenotype was observed ( Supplementary Fig. 8 ). We also investigated the role of Src, which is activated downstream of both integrin and syndecan receptors; Src signalling was similarly not required for dynamic catch bonds. These data, along with the timescales involved in force application between successive contacts and the observed dynamics of bond stiffening (that is, milliseconds), suggest that regulation of this rapid biological process is mechanical, rather than biochemical in nature. It has been well demonstrated that α 5 β 1 cooperates with Syn4 to mediate FA formation during cell spreading on fibronectin [15] , [16] , [57] . HSPGs also relate interstitial flow information to cytoskeletal remodelling through integrin-dependent FAK and ERK1/2 signalling [62] . Furthermore, it is commonplace to find integrin and syndecan-binding domains adjacent to one another within proteins (that is, fibronectin, vitronectin and fibrillin). However, the molecular basis for structural and functional connections between integrins and syndecans remains obscure [15] . Although a distinct ligand from fibronectin, Thy-1 shares an important similarity in which binding sites to both integrin and syndecan are present and adjacent. Based on the predicted three-dimensional structure of Thy-1 (no crystal structure exists), the syndecan-binding site (REKRK) is positioned on the face of the molecule opposite the integrin-binding site (RLD) [52] . The trimolecular complex model ( Fig. 4d ) may explain how Thy-1 physically bridges α 5 β 1 and Syn4 on the molecular level. Mechanistically, the trimolecular complex is formed in the absence of force, and this association is dictated by the synergistic effect of both α 5 β 1 and Syn4 receptors. The bond composition does not change on force application, but we are able to mechanically observe tightening of the co-receptor engagement (that is, bond stiffening) and the complex is strengthened (that is, catch bonds), supporting a mechanism whereby load sharing between the two receptors occurs once a threshold force is reached ( Fig. 4d ). We suggest that this threshold level is contributed by tightening deformation of the highly flexible GAG chains attached to the syndecan receptor. This mechanotransductory mechanism probably requires both receptors in a specific orientation and proximity within the plasma membrane, thereby allowing efficient signal propagation. It will be interesting for future studies to determine the differential downstream signalling responses at the molecular spatial- and sub-second time scales resulting from force-mediated co-receptor engagement and bond lifetime prolongation. Cells, proteins and antibodies K562 (ATCC, VA) and A375 cells (a kind gift of Jack Arbiser (Emory University, Atlanta, GA)) were cultured in DMEM supplemented with 10% fetal bovine serum and 100 μg ml −1 penicillin/streptomycin (Cellgro, VA). For BFP experiments, cells were washed with PBS containing 2 mM EDTA before resuspension in 10 mM HEPES containing 1% human serum albumin (HSA), 150 mM NaCl and 1 mM Mn 2+ . β 1 Integrin knockdown in K562 cells was performed using a lentiviral vector system specific to human β1 shRNA (NM-002211.3) [63] . Stable transfectants were selected in 2 μg G418 and sorted using FACS with fluorescein isothiocyanate (FITC)-conjugated anti-β 1 K-20 to undetectable expression levels by flow cytometry. For antibody-blocking experiments, anti-β 1 mAb AIIB2 (Developmental Studies Hybridoma Bank) or anti-Syn4 mAb 5G9 (Santa Cruz Biotechnology, Santa Cruz, CA) were used at concentrations of 20 μg ml −1 . For Syn4 siRNA knockdown, human Syn4 siRNA (SC-36588; Santa Cruz Biotechnology) or scrambled control siRNA (SC-37007; Santa Cruz Biotechnology) was transfected into K562 or A375 cells using the Amaxa Nucleofector system (Lonza, Switzerland) at 10 nM, and cells were used the following day for experimentation or verification of knockdown efficiency by flow cytometry. For HPSE treatments, cells were incubated with 1 mU HPSE III (heparitinase) in 10 mM HEPES containing 1% HSA, 150 mM NaCl, for 30 min at 37 °C before being washed and transferred to BFP experimental buffer. For native Thy-1 stretch assay, anti-human Thy-1 mAb 5E10 (BD Biosciences, NJ) was purchased. Recombinant α 5 β 1 –Fc was previously described [64] . Recombinant human Thy-1–Fc was purchased (Enzo Life Sciences, NY) or produced in-house. Thy-1–Fc fusion proteins were expressed in HEK293 cells and purified from culture supernatant using affinity chromatography with Protein A resin (Invitrogen, CA). Dynamin I-II inhibitor MiTMAB (Abcam, MA) and Src inhibitor PP2 (EMD Millipore, MA) were purchased and used at 10 and 20 μM, respectively. All reagents, if not specified, were purchased from Sigma-Aldrich (St Louis, MO). Cell spreading and FA analysis A375 cells were trypsinized, resuspended in soybean trypsin inhibitor and held in suspension for 30 min before plating on fibronectin (20 μg ml −1 ) or recombinant human Thy-1–Fc (Enzo, 50 μg ml −1 ) in serum-free DMEM. Samples were treated with 25 μM blebbistatin for 30 min and fixed with 4% formaldehyde in PBS after 90 min. For CHX experiments, cells were treated with 20 μg ml −1 CHX for 1 h beforetrypsinization and plated in the presence of CHX. After fixation for 10 min at 25 °C, samples were permeabilized with 0.2% Triton X-100 and blocked with 5% normal goat serum. Samples were then stained with mouse anti-Pxn 5H11 (1:200 dilution; Millipore, MA) and rabbit anti-FAK-pY397 (1:200 dilution; Invitrogen), followed by AlexaFluor 488 and 546 secondary antibodies (Invitrogen). Confocal fluorescence microscopy was performed using a Zeiss LSM 700 microscope with a × 63, 1.4 numerical aperture objective (Carl Zeiss, Inc.; Jena, Germany). Cells that were spread after 90 min were analysed. Pxn is used as the FA marker in this study, as its abundance in FAs is largely independent from myosin II activity [65] . This was used to generate a spatial mask to quantify and normalize local FAK activation as a function of myosin II activity, as has been done in previous studies [66] , [67] . An in-house built MATLAB script was used to quantify micrographs based on the morphometry and intensity of adhesions. After background subtraction, an intensity threshold was used to identify and mask structures based on the Pxn immunofluorescence signal. This mask was subsequently applied to both adhesion marker channels, and a ratiometric value for FAK-pY397 intensity/Pxn intensity was calculated on a per pixel basis. Masked pixels were also converted to binary sequence, and connected pixels were grouped into bins based on size and converted to μm 2 units. The average ratiometric value for single adhesion was calculated and compared with the area of single masked adhesion structures, or the average of all adhesions for an experimental group was calculated. Functionalization of glass beads Thy-1 was covalently modified with maleimide-PEG3500-NHS (molecular weight ~3,500 Da; JenKem, TX) in carbonate/bicarbonate buffer (pH 8.5). To coat maleimide-modified Thy-1 on glass beads, 2-μm (diameter) silanized borosilicate beads (Thermo Scientific) were first covalently coupled with mercapto-propyl-trimethoxy silane, followed by covalently linking to streptavidin-maleimide and modified Thy-1 in phosphate buffer (pH 6.8) ( Fig. 2a , left). After overnight incubation and resuspending in phosphate buffer with 1% HSA, beads were ready for immediate use in BFP experiments. For the Thy-1 stretch assay ( Supplementary Fig. 6a,b ), 5E10 mAb was immobilized on bead surfaces with the same protocol. To measure Thy-1 site density on the bead surface, Thy-1-coated beads were incubated with FITC-conjugated anti-Thy-1 mAb 5E10 (1:100 dilution, BD Biosciences) in phosphate buffer with 1% HSA at room temperature for 30 min. After washing in phosphate buffer, bead fluorescent intensities were measured using an Accuri C6 flow cytometer (BD Biosciences). The intensity results were compared with standard calibration beads (Quantum FITC-5 MESF; Bangs Laboratories, Inc., IN) to determine total number of molecules per bead using a manufacturer-provided calculating Excel form [68] . The site densities were calculated by dividing the total number of molecules per bead to the bead surface area, which was calculated from the bead diameters measured under the microscope (~3.5 μm). The cell surface expression of receptor molecules on K562 and A375 cells was measured in a similar manner. BFP assays Piezoelectric translator control and the image analysis were done on a personal computer using Labview programmes written in-house. Previously described adhesion frequency and force-clamp assays [30] were run as repeated cycles. In each cycle, the target was driven to approach and contact the probe with a 20-pN compressive force for a 0.5-s contact time that allowed for bond formation and then retracted for adhesion detection. During the retraction phase, an adhesion event was signified by tensile force ( Fig. 3a , blue and red traces), but no tensile force was detected in the no-adhesion event ( Fig. 3a , black trace). For the adhesion frequency assay, adhesion and no-adhesion events were enumerated to calculate an adhesion frequency in 50 repeated cycles for each probe and target pair. In the force-clamp assay, the target was held at a desired force to wait for bond dissociation and returned to the original position to complete the cycle. Lifetime was measured from the instant the force reached the desired level to the instant of bond dissociation ( Fig. 3a , blue and red traces) [30] . To ensure higher possibilities (>95%) for single-ligand bond events, we coated Thy-1 at a lower site density (~233 μm −2 ) in bond lifetime and molecular stiffness analysis than that (~898 μm −2 ) in adhesion frequency analysis. Furthermore, we specifically excluded events with multiple bond signatures from analysis (that is, events showing discrete slope decrease during force ramping phase or showing multiple-state unbinding in dissociation phase). For the stretch assay, the test cycle was similar to that in the force-clamp assay, except that the target was retracted at a constant velocity without stopping for a force clamp [29] . The force at which the bond dissociates was termed ‘rupture force’ ( Supplementary Fig. 6b ). Calculating bond fractions from adhesion frequency As described previously [69] , the adhesion frequency P a (subtract the nonspecific binding frequency P n from the total binding frequency P t , where P a = P t − P n ) is related to the average bond number ‹ n › by For adhesion mediated by dual receptor species, that is, integrin α 5 β 1 and Syn4, ‹ n › includes contributions from two independent Thy-1 bimolecular interactions, one to each species, denotes ‹ n α5β1 › and ‹ n Syn4 ›, respectively, and the Thy-1 trimolecular interaction to both species, denotes ‹ n α5β1+Syn4 ›. The total Thy-1 bond number ‹ n total › is calculated from the P a , measured from the Thy-1–K562 experiment under the no-treatment conditions and expressed as below where ‹ n α5β1 › and ‹ n Syn4 › are calculated from P a , measured from the same experimental setup using Syn4 and β 1 integrin knockdown K562 cells, respectively. As the same site density on Thy-1 beads were used for all experiments, and RNAi of Syn4 and β 1 integrin did not affect expression of the alternate receptor ( Supplementary Fig. 2c ), the molecule densities are kept as constants and not expected to bias the data interpretation. Calculating lifetimes for a mixed population of bonds For interactions mediated by single receptor species, α 5 β 1 or Syn4, their respective lifetimes, ‹ t α5β1 › or ‹ t Syn4 ›, were averaged from ensemble lifetimes measured. For interactions mediated by a mixed population of dual receptor species, the measured total bond lifetimes include contributions from two bimolecular interactions (α 5 β 1 and Syn4) and a trimolecular interaction (α 5 β 1 +Syn4). Assuming that both bimolecular bonds and the trimolecular bond unbind independently, the total average lifetime ‹ t total › can be expressed as where the subscripts identify the types of bonds. ‹ t α5β1 › and ‹ t Syn4 › were measured from the same experimental setup using Syn4 and β 1 integrin knockdown K562 cells. Stiffness analysis The stiffness of molecular bonds can be derived from BFP test cycles [29] , [70] . The ramping phase of each bond event ( Fig. 3b,c ) corresponds to a force versus extension curve ( Fig. 4a ), the slope of which is the stiffness of the system, including the cell (RBC plus K562) and the molecular complex serially linked. As such, the reciprocal of the system stiffness, 1/ k sys , equals the sum of the reciprocals of the cellular and molecular stiffness, 1/ k cell +1/ k mol [29] . The reasonable assumptions made here are: (1) the molecular complex can resist tension but not compression and (2) the cellular spring has the same value regardless of whether the cell surface is in tension or compression. The validity of these assumptions has been supported by the increased slope of the compressive segment than the tensile segment of the force versus extension curves ( Fig. 4a ). Here the extension was calculated as differential displacement between the BFP tracking system and the piezoelectric actuator feedback system. Thus, we estimated k cell and k sys from the respective slopes of the black and blue dashed lines, which are linear fits to the force versus extension curve segments for compression and tension, respectively ( Fig. 4a ). In non-stiffening events, only a single slope existed; thus, the molecular stiffness was calculated by k non-stiff = k mol 1 =1/(1/ k sys 1 −1/ k cell ). However, in stiffening events, a second slope (red dashed line) following the abrupt slope change, the kink (SP), was observed. The molecular stiffness before and after SP were calculated as k stiff 1 = k mol 1 =1/(1/ k sys 1 −1/ k cell ) and k stiff 2 = k mol 2 =1/(1/ k sys 2 −1/ k cell ), respectively. To discriminate two bond species (Thy-1–α 5 β 1 and Thy-1–Syn4) by their distinct bond stiffness, we fit a bimodal distribution from a histogram of an ensemble bond stiffness of the two receptor species. The histogram of measured k non-stiff was fitted with a double Gaussian kernel function: where N is the total fraction of molecular stiffness and k is molecular stiffness. k i , σ i and w i , ( i =1,2) are, respectively, the mean, s.d. and weight of the i th subpopulation. The weight w i represents an approximation to the total fraction of molecular stiffness of the i th sub-population. The fraction of each subpopulation is calculated by w i /( w 1 + w 2 ). The initial values are k 1 =0.6 and k 2 =0.9 pN nm −1 for Syn4 and α 5 β 1 bonds, respectively. The fitting and parameters calculations were analysed in GraphPad Prism 5.0b by the least squares fit method. How to cite this article : Fiore, V. F. et al . Dynamic catch of a Thy-1–α 5 β 1 +syndecan-4 trimolecular complex. Nat. Commun. 5:4886 doi: 10.1038/ncomms5886 (2014).